CARL lncRNA inhibits anoxia-induced mitochondrial fission and apoptosis in cardiomyocytes by impairing miR-539-dependent PHB2 downregulation Abnormal mitochondrial fission participates in the pathogenesis of many diseases. Long non-coding RNAs (lncRNAs) are emerging as new players in gene regulation, but how lncRNAs operate in the regulation of mitochondrial network is unclear. Here we report that a lncRNA, named cardiac apoptosis-related lncRNA (CARL), can suppress mitochondrial fission and apoptosis by targeting miR-539 and PHB2. The results show that PHB2 is able to inhibit mitochondrial fission and apoptosis. miR-539 is responsible for the dysfunction of PHB2 and regulates mitochondrial fission and apoptosis by targeting PHB2. Further, we show that CARL can act as an endogenous miR-539 sponge that regulates PHB2 expression, mitochondrial fission and apoptosis. Our present study reveals a model of mitochondrial fission regulation that is composed of CARL, miR-539 and PHB2. Modulation of their levels may provide a new approach for tackling apoptosis and myocardial infarction. Mitochondria constantly undergo fusion and fission that are necessary for the maintenance of organelle fidelity [1] . Mitochondrial dynamics have critical role in cell physiology. Strikingly, most recent studies have revealed that abnormal mitochondrial fusion and fission participate in the regulation of apoptosis. Mitochondrial fusion is able to inhibit apoptosis, while growing body of evidence reveals that the mitochondrial fission is necessary for initiation of apoptosis, although both events can be separate [1] , [2] , [3] , [4] , [5] , [6] , [7] . The prohibitin complex comprises two subunits, PHB1 and PHB2, and they are mainly localized in the mitochondrial inner membrane. These two proteins assemble into a ring-like macromolecular structure [8] , having a significant role in diverse intracellular processes such as mitochondrial biogenesis, cell cycle progression and aging [9] , [10] , as well as in many diseases like obesity, diabetes and cancer [11] . Also, PHB2 is an oestrogen receptor (ER)-binding protein and it represses transcriptional activation [12] . Recent findings suggest that PHB2 has an important role in regulating mitochondrial morphology. Loss of PHB2 results in accumulation of fragmented mitochondria in mouse embryonic fibroblasts (MEFs) and HeLa cells [13] , [14] . PHB2 is abundantly expressed in cardiomyocytes under physiological condition [15] . However, it is not yet clear whether PHB2 participates in the regulation of mitochondrial dynamics in cardiomyocytes. MicroRNAs (miRNAs) are a class of small non-coding RNAs that bind to the 3′-untranslated region (3′-UTR) of mRNAs, thereby inhibiting mRNA translation or promoting mRNA degradation [16] . Growing evidence has demonstrated that miRNAs can have a significant role in the regulation of development, differentiation, proliferation and apoptosis [17] . Long non-coding RNAs (lncRNAs) are transcribed RNA molecules >200 nucleotides in length, with no significant protein-coding potential. LncRNAs have many specific functional features and are involved in many diverse biological processes in cells, such as RNA processing [18] , modulation of apoptosis and invasion [19] , marker of cell fate [20] and chromatin modification [21] and so on. In addition, lncRNAs can act as a competing endogenous RNA in mouse and human myoblasts [22] . However, it is not yet clear whether lncRNA is involved in the regulation of mitochondrial fission. Our present work reveals that PHB2 has a key role in maintaining the homeostasis of mitochondrial dynamics. PHB2 is negatively regulated by miR-539 that can affect mitochondrial fission and apoptosis. Moreover, our study further suggests that cardiac apoptosis-related lncRNA (CARL) can directly bind to miR-539 and participates in the regulation of mitochondrial network and apoptosis through the miR-539/PHB2 pathway. Our data shed new light on the understanding of the interaction between lncRNA and miRNA in molecular regulation of mitochondrial network. PHB2 is able to inhibit mitochondrial fission and apoptosis Abnormal mitochondrial fusion and fission participate in the regulation of apoptosis. PHB2 is mainly localized in the mitochondrial inner membrane and has an important role in regulating mitochondrial morphology. Recent findings suggest that loss of PHB2 results in accumulation of fragmented mitochondria in MEFs and HeLa cells [13] , [14] . However, the role of PHB2 in mitochondrial dynamics in the heart remains unknown. To test whether PHB2 participates in the regulation of mitochondrial fission in cardiomyocytes, we treated cardiomyocytes with anoxia to induce apoptosis and mitochondrial fission. The expression levels of PHB2 in mitochondria were downregulated after anoxia treatment ( Fig. 1a ). The cells underwent mitochondrial fission upon anoxic treatment ( Fig. 1b ). We then tested whether PHB2 is related to the occurrence of mitochondrial fission. Enforced expression of PHB2 attenuated mitochondrial fission ( Fig. 1c,d ) and apoptosis ( Fig. 1e and Supplementary Fig. 1a ) induced by anoxia. Myocardial ischaemia led to a reduction of PHB2 levels in mitochondria ( Fig. 1f ). To understand the role of PHB2 in myocardial infarction (INF), we used the ischaemia/reperfusion (I/R) model. I/R also induced a reduction of PHB2 levels in mitochondria ( Fig. 1g ). Enforced expression of PHB2 ( Supplementary Fig. 1b ) resulted in a reduction in mitochondrial fission and apoptosis ( Fig. 1h ), and infarct sizes ( Fig. 1i ) upon I/R. Cardiac function was also ameliorated ( Supplementary Fig. 1c ). Further, knockdown of PHB2 ( Supplementary Fig. 2a ) resulted in an increase in mitochondrial fission ( Supplementary Fig. 2b ) and infarct sizes ( Supplementary Fig. 2c ) upon I/R. These data suggest that PHB2 can inhibit mitochondrial fission, apoptosis and myocardial INF. 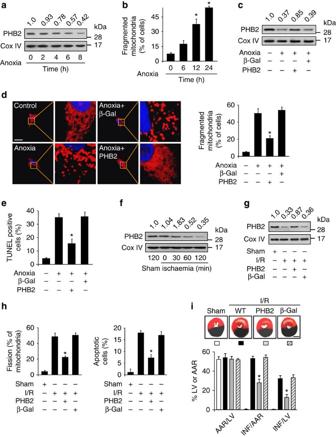Figure 1: PHB2 is able to inhibit mitochondrial fission and apoptosis. (a) Anoxia induces a reduction of PHB2 levels in mitochondria. Cardiomyocytes were exposed to anoxia. PHB2 levels were analysed by immunoblot;n=3. (b) Anoxia induces mitochondrial fission. The cells with fragmented mitochondria were counted. Data are shown as mean±s.e.m. of three independent experiments. *P<0.05 versus control in Student’st-test. (c) Enforced expression of PHB2 restores the reduction of PHB2 levels induced by anoxia in mitochondria. Cardiomyocytes were infected with adenoviral PHB2 and β-gal, then exposed to anoxia. PHB2 levels were analysed by immunoblot;n=3. (d,e) Enforced expression of PHB2 prevents mitochondrial fission and apoptosis induced by anoxia. Cardiomyocytes were treated as described inc, the cells were stained with mitotracker-red (d, left panel); scale bar, 20 μm. The cells with fragmented mitochondria were counted (d, right panel). Apoptosis was analysed by TUNEL assay (e). Data are shown as mean±s.e.m. of three independent experiments. *P<0.05 versus anoxia alone in one-way analysis of variance. (f) The levels of PHB2 are decreased in myocardial ischaemia. Mice were induced to undergo cardiac ischaemia as described in methods. PHB2 levels were analysed by immunoblot (n=3). (g) Enforced expression of PHB2 restores the levels of PHB2 upon I/R. Intracoronary delivery of adenoviral constructs and I/R are described in Methods. PHB2 levels were analysed by immunoblot (n=4). (h) Enforced expression of PHB2 attenuates mitochondrial fission and apoptosis upon I/R. The mice were treated as described ing. Counting of the fragmented mitochondria by EM and apoptosis by TUNEL were shown. Data are shown as mean±s.e.m. of four independent experiments. *P<0.05 versus I/R alone in one-way analysis of variance. (i) Enforced expression of PHB2 attenuates myocardial INF sizes. The upper panels are myocardial representative photos of midventricular myocardial slices. The low panel shows infarct sizes. Area-at-risk (AAR), left ventricle (LV), infarct area (INF). Data are shown as mean±s.e.m. of six independent experiments. *P<0.05 versus I/R in one-way analysis of variance. Figure 1: PHB2 is able to inhibit mitochondrial fission and apoptosis. ( a ) Anoxia induces a reduction of PHB2 levels in mitochondria. Cardiomyocytes were exposed to anoxia. PHB2 levels were analysed by immunoblot; n =3. ( b ) Anoxia induces mitochondrial fission. The cells with fragmented mitochondria were counted. Data are shown as mean±s.e.m. of three independent experiments. * P <0.05 versus control in Student’s t- test. ( c ) Enforced expression of PHB2 restores the reduction of PHB2 levels induced by anoxia in mitochondria. Cardiomyocytes were infected with adenoviral PHB2 and β-gal, then exposed to anoxia. PHB2 levels were analysed by immunoblot; n =3. ( d , e ) Enforced expression of PHB2 prevents mitochondrial fission and apoptosis induced by anoxia. Cardiomyocytes were treated as described in c , the cells were stained with mitotracker-red ( d , left panel); scale bar, 20 μm. The cells with fragmented mitochondria were counted ( d , right panel). Apoptosis was analysed by TUNEL assay ( e ). Data are shown as mean±s.e.m. of three independent experiments. * P <0.05 versus anoxia alone in one-way analysis of variance. ( f ) The levels of PHB2 are decreased in myocardial ischaemia. Mice were induced to undergo cardiac ischaemia as described in methods. PHB2 levels were analysed by immunoblot ( n =3). ( g ) Enforced expression of PHB2 restores the levels of PHB2 upon I/R. Intracoronary delivery of adenoviral constructs and I/R are described in Methods. PHB2 levels were analysed by immunoblot ( n =4). ( h ) Enforced expression of PHB2 attenuates mitochondrial fission and apoptosis upon I/R. The mice were treated as described in g . Counting of the fragmented mitochondria by EM and apoptosis by TUNEL were shown. Data are shown as mean±s.e.m. of four independent experiments. * P <0.05 versus I/R alone in one-way analysis of variance. ( i ) Enforced expression of PHB2 attenuates myocardial INF sizes. The upper panels are myocardial representative photos of midventricular myocardial slices. The low panel shows infarct sizes. Area-at-risk (AAR), left ventricle (LV), infarct area (INF). Data are shown as mean±s.e.m. of six independent experiments. * P <0.05 versus I/R in one-way analysis of variance. Full size image miR-539 participates in the regulation of PHB2 expression miRNA is able to suppress gene expression. To explore the underlying mechanism by which PHB2 is downregulated upon anoxia and I/R treatment, we tested whether PHB2 is regulated by miRNA. We first analysed the 3′-UTR of PHB2 using the target scan programme ( http://www.targetscan.org/ ) and found several potential miRNAs (miR-539, miR-323-5p, miR-3062 and miR-325). All of them have evolutionarily conserved binding sites in the PHB2 3′-UTR. In order to identify the genuine miRNA that regulates PHB2, we used quantitative reverse transcription-PCR (qRT-PCR) to detect miRNA levels in response to anoxia treatment. Among four miRNAs, miR-539 was significantly upregulated upon anoxia ( Supplementary Fig. 3a , Fig. 2a,b ) that promoted us to focus on its function. We used several approaches to explore whether PHB2 expression can be regulated by miR-539. To this end, we first tested whether overexpress or knockdown of miR-539 can alter the expression of endogenous PHB2. Enforced expression of miR-539 led to a reduction of PHB2 levels in mitochondria ( Fig. 2c ), while administration of miR-539 antagomir could attenuate the decrease of PHB2 levels in response to anoxia ( Fig. 2d ). To understand whether the effect of miR-539 on PHB2 is specific, we then used the Target Protector technology [23] . The inhibitory effect of miR-539 on PHB2 expression was reduced in the presence of the target protector ( Fig. 2e ). PHB2 downregulation was attenuated by the target protector in response to anoxia ( Fig. 2f ). These results indicate that miR-539 can specifically regulate PHB2. 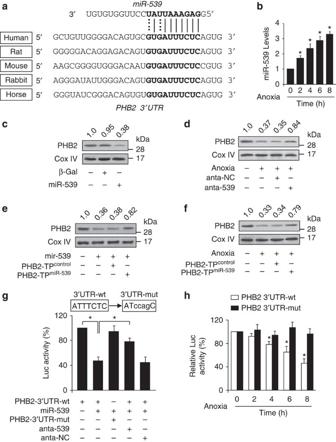Figure 2: miR-539 participates in the regulation of PHB2 expression. (a) Putative miR-539-binding site in the 3′-UTR region of PHB2. (b) Cardiomyocytes were exposed to anoxia. miR-539 levels were analysed by qRT-PCR. Data are shown as mean±s.e.m. of four independent experiments. *P<0.05 versus control in Student’st-test. (c) miR-539 suppresses the expression of PHB2. Cardiomyocytes were infected with adenoviral miR-539 or β-gal. The levels of PHB2 were analysed by immunoblot (n=3). (d) Knockdown of miR-539 attenuates the decrease in PHB2 levels upon anoxia. Cardiomyocytes were transfected with miR-539 antagomir (anta-539) or the antagomir-negative control (anta-NC),and then exposed to anoxia. The levels of PHB2 were analysed by immunoblot (n=3). (e) PHB2 target protector attenuates the reduction of PHB2 induced by miR-539. Cardiomyocytes were infected with adenoviral miR-539, and then transfected with the target protector (PHB2-TPmiR-539) or the control (PHB2-TPcontrol). PHB2 levels were analysed by immunoblot (n=3). (f) PHB2 target protector attenuates the reduction of PHB2 upon anoxia. Cardiomyocytes were transfected with the PHB2-TPmiR-539or PHB2-TPcontrol, and then exposed to anoxia. The levels of PHB2 in mitochondria were analysed by immunoblot (n=3). (g) miR-539 suppresses PHB2 translation. HEK293 cells were transfected with the luciferase constructs of the WT PHB2-3′-UTR (PHB2–3′-UTR-wt) or the mutated PHB2–3′-UTR (PHB2-3′-UTR-mut), along with the expression plasmid for miR-539, anta-539 or anta-NC. The luciferase activity was analysed. Data are shown as mean±s.e.m. of three independent experiments. *P<0.05 in one-way analysis of variance. (h) Anoxia can attenuate the translational activity of WT PHB2–3′-UTR but not the mutated PHB2–3′-UTR. Cardiomyocytes were transfected with the luciferase constructs of WT PHB2-3′-UTR-wt or the PHB2-3′-UTR-mut, then treated with anoxia, and then harvested at the indicated time for the luciferase assay. Data are shown as mean±s.e.m. of three independent experiments. *P<0.05 versus control in Student’st-test. Figure 2: miR-539 participates in the regulation of PHB2 expression. ( a ) Putative miR-539-binding site in the 3′-UTR region of PHB2. ( b ) Cardiomyocytes were exposed to anoxia. miR-539 levels were analysed by qRT-PCR. Data are shown as mean±s.e.m. of four independent experiments. * P <0.05 versus control in Student’s t- test. ( c ) miR-539 suppresses the expression of PHB2. Cardiomyocytes were infected with adenoviral miR-539 or β-gal. The levels of PHB2 were analysed by immunoblot ( n =3). ( d ) Knockdown of miR-539 attenuates the decrease in PHB2 levels upon anoxia. Cardiomyocytes were transfected with miR-539 antagomir (anta-539) or the antagomir-negative control (anta-NC),and then exposed to anoxia. The levels of PHB2 were analysed by immunoblot ( n =3). ( e ) PHB2 target protector attenuates the reduction of PHB2 induced by miR-539. Cardiomyocytes were infected with adenoviral miR-539, and then transfected with the target protector (PHB2-TP miR-539 ) or the control (PHB2-TP control ). PHB2 levels were analysed by immunoblot ( n =3). ( f ) PHB2 target protector attenuates the reduction of PHB2 upon anoxia. Cardiomyocytes were transfected with the PHB2-TP miR-539 or PHB2-TP control , and then exposed to anoxia. The levels of PHB2 in mitochondria were analysed by immunoblot ( n =3). ( g ) miR-539 suppresses PHB2 translation. HEK293 cells were transfected with the luciferase constructs of the WT PHB2-3′-UTR (PHB2–3′-UTR-wt) or the mutated PHB2–3′-UTR (PHB2-3′-UTR-mut), along with the expression plasmid for miR-539, anta-539 or anta-NC. The luciferase activity was analysed. Data are shown as mean±s.e.m. of three independent experiments. * P <0.05 in one-way analysis of variance. ( h ) Anoxia can attenuate the translational activity of WT PHB2–3′-UTR but not the mutated PHB2–3′-UTR. Cardiomyocytes were transfected with the luciferase constructs of WT PHB2-3′-UTR-wt or the PHB2-3′-UTR-mut, then treated with anoxia, and then harvested at the indicated time for the luciferase assay. Data are shown as mean±s.e.m. of three independent experiments. * P <0.05 versus control in Student’s t- test. Full size image We used the luciferase assay system to test whether miR-539 can influence the translation of PHB2. As shown in Fig. 2g , the wild-type (WT) 3′-UTR of PHB2 exhibited a low translation level in the presence of miR-539, whereas the mutated 3′-UTR did not show a significant response to miR-539. miR-539 in the presence of its antagomir induced a less effect on PHB2 translation, suggesting that the inhibitory effect of miR-539 is specific. We detected the translation ability of PHB2 in response to anoxia. The WT 3′-UTR of PHB2 but not the mutated 3′-UTR presented a reduced luciferase activity ( Fig. 2h ). Taken together, it appears that PHB2 is a specific target of miR-539. miR-539 can provoke mitochondrial fission and apoptosis We explored the functional role of miR-539 in mitochondrial fission and apoptosis. The antagomir of miR-539 efficiently attenuated the miR-539 levels ( Fig. 3a ) and mitochondrial fission induced by anoxia ( Fig. 3b ). Concomitantly, apoptosis was reduced in the presence of miR-539 antagomir ( Fig. 3c ). These data indicate that miR-539 can promote mitochondrial fission and apoptosis. 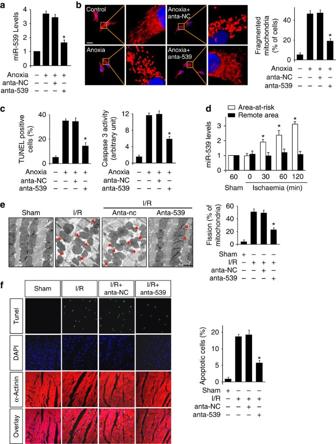Figure 3: miR-539 provokes mitochondrial fission programme. (a) miR-539 antagomir inhibits the elevation of miR-539 levels upon anoxia. Cardiomyocytes were transfected with anta-539 or anta-NC, then exposed to anoxia. Cells were harvested for qRT-PCR analysis of miR-539 levels. Data are shown as mean±s.e.m. of three independent experiments. *P<0.05 versus anoxia alone in one-way analysis of variance. (b) Knockdown of miR-539 prevents mitochondrial fission induced by anoxia. Cardiomyocytes were treated as described ina, the cells with fragmented mitochondria were counted. Data are shown as mean±s.e.m. of three independent experiments. *P<0.05 versus anoxia alone in one-way analysis of variance. (c) Knockdown of miR-539 prevents apoptosis induced by anoxia. Cardiomyocytes were treated as described inb. Apoptosis was analysed by TUNEL assay (left panel). The caspase-3 activity was analysed by using an Apo-ONE Homogeneous Caspase-3/7 assay kit (right panel). Data are shown as mean±s.e.m. of four independent experiments. *P<0.05 versus anoxia alone in one-way analysis of variance. (d) miR-539 levels during myocardial ischaemia. Mice were induced to undergo cardiac ischaemia. AAR and the remote area were prepared for qRT-PCR analysis of miR-539 levels. Data are shown as mean±s.e.m. of five independent experiments. *P<0.05 versus sham in Student’st-test. (e) Knockdown of miR-539 attenuates mitochondrial fission upon I/R. I.v. injections of miR-539 antagomir and I/R were performed as described in Methods. Representative EM images of heart tissue were shown in left panel; scale bar, 1 μm. Counting of the fragmented mitochondria were shown in right panel. Data are shown as mean±s.e.m. of six independent experiments. *P<0.05 versus I/R alone in one-way analysis of variance. (f) Knockdown of miR-539 inhibits cardiomyocyte apoptosis induced by I/R. The mice were treated as described ine. Apoptosis was analysed by TUNEL assay. Data are shown as mean±s.e.m. of six independent experiments. *P<0.05 versus I/R alone in one-way analysis of variance. Figure 3: miR-539 provokes mitochondrial fission programme. ( a ) miR-539 antagomir inhibits the elevation of miR-539 levels upon anoxia. Cardiomyocytes were transfected with anta-539 or anta-NC, then exposed to anoxia. Cells were harvested for qRT-PCR analysis of miR-539 levels. Data are shown as mean±s.e.m. of three independent experiments. * P <0.05 versus anoxia alone in one-way analysis of variance. ( b ) Knockdown of miR-539 prevents mitochondrial fission induced by anoxia. Cardiomyocytes were treated as described in a , the cells with fragmented mitochondria were counted. Data are shown as mean±s.e.m. of three independent experiments. * P <0.05 versus anoxia alone in one-way analysis of variance. ( c ) Knockdown of miR-539 prevents apoptosis induced by anoxia. Cardiomyocytes were treated as described in b . Apoptosis was analysed by TUNEL assay (left panel). The caspase-3 activity was analysed by using an Apo-ONE Homogeneous Caspase-3/7 assay kit (right panel). Data are shown as mean±s.e.m. of four independent experiments. * P <0.05 versus anoxia alone in one-way analysis of variance. ( d ) miR-539 levels during myocardial ischaemia. Mice were induced to undergo cardiac ischaemia. AAR and the remote area were prepared for qRT-PCR analysis of miR-539 levels. Data are shown as mean±s.e.m. of five independent experiments. * P <0.05 versus sham in Student’s t- test. ( e ) Knockdown of miR-539 attenuates mitochondrial fission upon I/R. I.v. injections of miR-539 antagomir and I/R were performed as described in Methods. Representative EM images of heart tissue were shown in left panel; scale bar, 1 μm. Counting of the fragmented mitochondria were shown in right panel. Data are shown as mean±s.e.m. of six independent experiments. * P <0.05 versus I/R alone in one-way analysis of variance. ( f ) Knockdown of miR-539 inhibits cardiomyocyte apoptosis induced by I/R. The mice were treated as described in e . Apoptosis was analysed by TUNEL assay. Data are shown as mean±s.e.m. of six independent experiments. * P <0.05 versus I/R alone in one-way analysis of variance. Full size image To understand the pathophysiological role of miR-539, we detected whether miR-539 is involved in the pathogenesis of myocardial INF in the animal model. miR-539 was elevated in response to ischaemia ( Fig. 3d ). Knockdown of miR-539 by antagomir delivery in vivo ( Supplementary Fig. 3b ) resulted in a reduction in mitochondrial fission ( Fig. 3e ), apoptosis ( Fig. 3f ) and infarct sizes ( Supplementary Fig. 3c ) upon I/R. The cardiac function was ameliorated by knockdown of miR-539 ( Supplementary Fig. 3d ). Thus, miR-539 has a functional role in mitochondrial fission, apoptosis and myocardial INF. miR-539 targets PHB2 To know how miR-539 elicits its effect on mitochondrial fission and apoptotic programme, we tested whether PHB2 is a downstream target of miR-539. PHB2-siRNA (small interfering RNA) could significantly reduce PHB2 expression levels ( Fig. 4a ). Knockdown of miR-539 inhibited anoxia-induced mitochondrial fission and apoptosis; however, this inhibitory effect was attenuated by knockdown of PHB2 ( Fig. 4b,c ). The target protector of PHB2 could inhibit mitochondrial fission and apoptosis induced by anoxia ( Fig. 4d ). In the animal model, the target protector of PHB2 ( Supplementary Fig. 4a ) also attenuated mitochondrial fission ( Fig. 4e , upper panel), apoptosis ( Fig. 4e , low panel) and infarct sizes ( Supplementary Fig. 4b ) upon I/R. These data suggest that miR-539 and PHB2 are functionally linked. 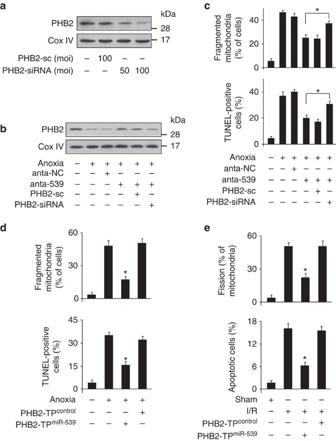Figure 4: miR-539 regulates mitochondrial fission and apoptosis through targeting PHB2. (a) Knockdown of PHB2 expression by PHB2-siRNA constructs. Cardiomyocytes were infected with adenoviral PHB2-siRNA or its scramble form (PHB2-sc) at the indicated moi. PHB2 levels in mitochondria were analysed by immunoblot. (b,c) Knockdown of PHB2 attenuates the inhibitory effect of miR-539 antagomir on mitochondrial fission and apoptosis upon anoxia. Cardiomyocytes were infected with adenoviral PHB2-siRNA or its scramble form, transfected with anta-539 or anta-NC and exposed to anoxia. Cells were harvested for the analysis of PHB2 expression levels (b), mitochondrial fission and apoptosis (c). Data are shown as mean±s.e.m. of three independent experiments. *P<0.05 in one-way analysis of variance. (d) PHB2 target protector inhibits mitochondrial fission and apoptosis induced by anoxia. Cardiomyocytes were transfected with the target protector (PHB2-TPmiR-539) or the control (PHB2-TPcontrol), and then exposed to anoxia. Mitochondrial fission (upper panel) and apoptosis (low panel) were analysed. Data are shown as mean±s.e.m. of three independent experiments. *P<0.05 versus anoxia alone in one-way analysis of variance. (e) PHB2 target protector attenuates mitochondrial fission and apoptosis upon I/R. Mice were treated as described in Methods. Mitochondrial fission (upper panel) and the quantitative analysis of apoptotic (low panel) were shown. Data are shown as mean±s.e.m. of five independent experiments. *P<0.05 versus I/R in one-way analysis of variance. Figure 4: miR-539 regulates mitochondrial fission and apoptosis through targeting PHB2. ( a ) Knockdown of PHB2 expression by PHB2-siRNA constructs. Cardiomyocytes were infected with adenoviral PHB2-siRNA or its scramble form (PHB2-sc) at the indicated moi. PHB2 levels in mitochondria were analysed by immunoblot. ( b , c ) Knockdown of PHB2 attenuates the inhibitory effect of miR-539 antagomir on mitochondrial fission and apoptosis upon anoxia. Cardiomyocytes were infected with adenoviral PHB2-siRNA or its scramble form, transfected with anta-539 or anta-NC and exposed to anoxia. Cells were harvested for the analysis of PHB2 expression levels ( b ), mitochondrial fission and apoptosis ( c ). Data are shown as mean±s.e.m. of three independent experiments. * P <0.05 in one-way analysis of variance. ( d ) PHB2 target protector inhibits mitochondrial fission and apoptosis induced by anoxia. Cardiomyocytes were transfected with the target protector (PHB2-TP miR-539 ) or the control (PHB2-TP control ), and then exposed to anoxia. Mitochondrial fission (upper panel) and apoptosis (low panel) were analysed. Data are shown as mean±s.e.m. of three independent experiments. * P <0.05 versus anoxia alone in one-way analysis of variance. ( e ) PHB2 target protector attenuates mitochondrial fission and apoptosis upon I/R. Mice were treated as described in Methods. Mitochondrial fission (upper panel) and the quantitative analysis of apoptotic (low panel) were shown. Data are shown as mean±s.e.m. of five independent experiments. * P <0.05 versus I/R in one-way analysis of variance. Full size image CARL is able to regulate miR-539 expression and activity How is miR-539 expression regulated under the pathological condition? Recent studies have suggested that lncRNAs may act as endogenous sponge RNA to interact with miRNAs and influence the expression of miRNA [22] , [24] , [25] . To explore the underlying mechanism responsible for miR-539 upregulation in response to anoxia treatment, we tested whether lncRNA can be involved in the apoptotic pathway of anoxia treatment. We screened 100 lncRNAs with high expression levels in heart from a result of lncRNA array performed by Fantom company. We carried out qRT-PCR to detect lncRNAs levels upon anoxia treatment. Among those lncRNAs, four lncRNAs were substantially reduced ( Fig. 5a and Supplementary Table 1 ). To understand which lncRNA is involved in the regulation of miR-539, we separately knocked down the four lncRNAs by siRNA technology. The results showed that only knockdown of AK017121 (UCSC Genome Browser on Mouse, 2011 Assembly) which we named CARL, led to an increase of miR-539 expression levels ( Fig. 5b ), and the other three lncRNAs had no effect on the miR-539 expression ( Supplementary Fig. 5a ). So we speculate that CARL might serve as sponge of miR-539. The expression level of CARL is more than twice than that of miR-539 in mouse heart ( Supplementary Fig. 5b ) and CARL is also widely expressed in various tissues ( Supplementary Fig. 5c ). To know whether CARL can affect miR-539 activity, we constructed miR-539 sensor. The miR-539 sensor construct contains a perfect miR-539 target and reduced luciferase activity of sensor indicates the induction of miR-539 activity. Our results showed that the luciferase activity of miR-539 sensor was decreased in cells treated with CARL-siRNA ( Fig. 5c ), suggesting the induction of miR-539 activity. Enforced expression of CARL ( Fig. 5d , low panel) induced a reduction in miR-539 expression ( Fig. 5d , upper panel) and activity ( Fig. 5e and Supplementary Fig. 5d ). To further test whether CARL may act as a sponge for miR-539, we transfected the cells with miR-539 sensor luciferase reporter, and adenoviral miR-539, CARL or β-galactosidase (β-gal) ( Supplementary Fig. 5e ). The luciferase activity showed that CARL counteracted the effect of miR-539 ( Fig. 5f ), suggesting that CARL is a functional sponge for miR-539. Taken together, these data suggest that CARL is able to regulate miR-539 levels and activity. 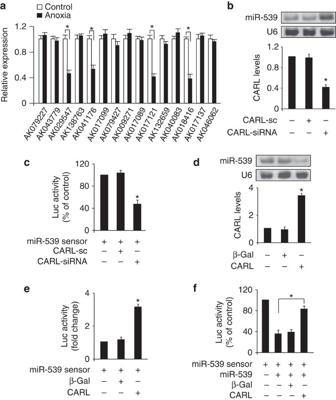Figure 5: CARL can regulate miR-539 expression and activity. (a) LncRNAs expression levels upon treatment with anoxia. Cardiomyocytes were untreated (control) or treated with anoxia for 24 h. LncRNAs chosen from Fantom company were analysed by qRT-PCR. Data are shown as mean±s.e.m. of four independent experiments. *P<0.05 in Student’st-test. (b) Knockdown of CARL induces the increase of miR-539 expression levels. Cardiomyocytes were infected with adenoviral CARL-siRNA (CARL-siRNA) and its scramble form (CARL-sc). miR-539 levels were analysed by northern blot (upper panel) and CARL levels were analysed by real-time PCR (low panel). Data are shown as mean±s.e.m. of three independent experiments. *P<0.05 versus control in one-way analysis of variance. (c) Knockdown of CARL induces miR-539 activity. Cardiomyocytes were infected with adenoviral CARL-siRNA and its scramble form, then transfected with miR-539 sensor. Luciferase activity was analysed. Data are shown as mean±s.e.m. of three independent experiments. *P<0.05 versus miR-539 sensor alone in one-way analysis of variance. (d) Enforced expression of CARL reduces the expression levels of miR-539. Cardiomyocytes were infected with adenoviral CARL or β-gal. miR-539 levels were analysed by northern blot (upper panel) and CARL levels were analysed by real-time PCR (low panel). Data are shown as mean±s.e.m. of three independent experiments. *P<0.05 versus control in one-way analysis of variance. (e) CARL reduces miR-539 activity. Cardiomyocytes were infected with adenoviral CARL or β-gal, then transfected with miR-539 sensor. Luciferase activity was analysed. Data are shown as mean±s.e.m. of three independent experiments. *P<0.05 versus miR-539 sensor alone in one-way analysis of variance. (f) CARL acts as a sponge for miR-539. Cardiomyocytes were infected with adenoviral miR-539, CARL or β-gal, then transfected with miR-539 sensor. Luciferase activity was analysed. Data are shown as mean±s.e.m. of three independent experiments. *P<0.05 in one-way analysis of variance. Figure 5: CARL can regulate miR-539 expression and activity. ( a ) LncRNAs expression levels upon treatment with anoxia. Cardiomyocytes were untreated (control) or treated with anoxia for 24 h. LncRNAs chosen from Fantom company were analysed by qRT-PCR. Data are shown as mean±s.e.m. of four independent experiments. * P <0.05 in Student’s t- test. ( b ) Knockdown of CARL induces the increase of miR-539 expression levels. Cardiomyocytes were infected with adenoviral CARL-siRNA (CARL-siRNA) and its scramble form (CARL-sc). miR-539 levels were analysed by northern blot (upper panel) and CARL levels were analysed by real-time PCR (low panel). Data are shown as mean±s.e.m. of three independent experiments. * P <0.05 versus control in one-way analysis of variance. ( c ) Knockdown of CARL induces miR-539 activity. Cardiomyocytes were infected with adenoviral CARL-siRNA and its scramble form, then transfected with miR-539 sensor. Luciferase activity was analysed. Data are shown as mean±s.e.m. of three independent experiments. * P <0.05 versus miR-539 sensor alone in one-way analysis of variance. ( d ) Enforced expression of CARL reduces the expression levels of miR-539. Cardiomyocytes were infected with adenoviral CARL or β-gal. miR-539 levels were analysed by northern blot (upper panel) and CARL levels were analysed by real-time PCR (low panel). Data are shown as mean±s.e.m. of three independent experiments. * P <0.05 versus control in one-way analysis of variance. ( e ) CARL reduces miR-539 activity. Cardiomyocytes were infected with adenoviral CARL or β-gal, then transfected with miR-539 sensor. Luciferase activity was analysed. Data are shown as mean±s.e.m. of three independent experiments. * P <0.05 versus miR-539 sensor alone in one-way analysis of variance. ( f ) CARL acts as a sponge for miR-539. Cardiomyocytes were infected with adenoviral miR-539, CARL or β-gal, then transfected with miR-539 sensor. Luciferase activity was analysed. Data are shown as mean±s.e.m. of three independent experiments. * P <0.05 in one-way analysis of variance. Full size image CARL is able to directly bind to miR-539 in vivo To understand the mechanism by which CARL regulates the levels of miR-539, we tested whether CARL can interact with miR-539. We compared the sequences of CARL with that of miR-539 using the bioinformatics programme RNAhybrid and noticed that CARL contains a binding site of miR-539 ( Fig. 6a ). We produced a luciferase construct of CARL (Luc-CARL-wt) and a mutated form (Luc-CARL-mut) ( Fig. 6b ). Luciferase assay revealed that miR-539 could suppress the luciferase activity of CARL, but it had less effect on the mutated form of CARL ( Fig. 6c ). These results revealed that CARL may interact with miR-539 by this putative binding site. 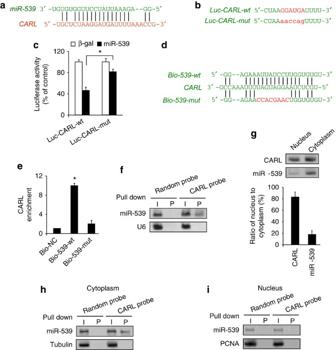Figure 6: Interaction between CARL and miR-539. (a) CARL RNA contains a site complementary to miR-539. (b) Luciferase constructs. miR-539-binding site in CARL RNA WT form (Luc-CARL-wt) and the mutated form (Luc-CARL-mut) are shown. (c) Luciferase assay. HEK293 cells were infected with adenoviral miR-539 or β-gal, then transfected with the luciferase constructs of Luc-CARL-wt or Luc-CARL-mut. The luciferase activity was analysed. Data are shown as mean±s.e.m. of three independent experiments. *P<0.05 in one-way analysis of variance. (d) WT and the mutated form of miR-539 sequence are shown. (e) CARL is associated with miR-539. Cardiomyocytes were transfected with biotinylated WT miR-539 (Bio-539-wt) or biotinylated mutant miR-539 (Bio-539-mut). A biotinylated miRNA that is not complementary to CARL was used as a NC (Bio-NC). 48 h after transfection, cells were harvested for biotin-based pulldown assay. CARL expression levels were analysed by real-time PCR. Data are shown as mean±s.e.m. of four independent experiments. *P<0.05 versus Bio-NC in one-way analysis of variance. (f) miR-539 is associated with CARL. miR-539 was pulled down by the CARL probe or random probe. The levels of miR-539 were analysed by northern blot. I, input (10% samples were loaded); P, pellet (100% samples were loaded). (g) Detection in nuclear or cytoplasmic fractions of CARL and miR-539 in cardiomyocytes. The levels of CARL and miR-539 were analysed by northern blot. (h,i) miR-539 could be pulled down by the CARL probe in the cytoplasm (h) but not in the nucleus (i). Cells were collected for the analysis of miR-539 by northern blot or by immunoblot with the cellular fractions of cytoplasm or nucleus. I, input (10% samples were loaded); P, pellet (100% samples were loaded). Proliferating cell nuclear antigen (PCNA) is a nuclear marker. Tubulin is a cytoplasmic marker. Figure 6: Interaction between CARL and miR-539. ( a ) CARL RNA contains a site complementary to miR-539. ( b ) Luciferase constructs. miR-539-binding site in CARL RNA WT form (Luc-CARL-wt) and the mutated form (Luc-CARL-mut) are shown. ( c ) Luciferase assay. HEK293 cells were infected with adenoviral miR-539 or β-gal, then transfected with the luciferase constructs of Luc-CARL-wt or Luc-CARL-mut. The luciferase activity was analysed. Data are shown as mean±s.e.m. of three independent experiments. * P <0.05 in one-way analysis of variance. ( d ) WT and the mutated form of miR-539 sequence are shown. ( e ) CARL is associated with miR-539. Cardiomyocytes were transfected with biotinylated WT miR-539 (Bio-539-wt) or biotinylated mutant miR-539 (Bio-539-mut). A biotinylated miRNA that is not complementary to CARL was used as a NC (Bio-NC). 48 h after transfection, cells were harvested for biotin-based pulldown assay. CARL expression levels were analysed by real-time PCR. Data are shown as mean±s.e.m. of four independent experiments. * P <0.05 versus Bio-NC in one-way analysis of variance. ( f ) miR-539 is associated with CARL. miR-539 was pulled down by the CARL probe or random probe. The levels of miR-539 were analysed by northern blot. I, input (10% samples were loaded); P, pellet (100% samples were loaded). ( g ) Detection in nuclear or cytoplasmic fractions of CARL and miR-539 in cardiomyocytes. The levels of CARL and miR-539 were analysed by northern blot. ( h , i ) miR-539 could be pulled down by the CARL probe in the cytoplasm ( h ) but not in the nucleus ( i ). Cells were collected for the analysis of miR-539 by northern blot or by immunoblot with the cellular fractions of cytoplasm or nucleus. I, input (10% samples were loaded); P, pellet (100% samples were loaded). Proliferating cell nuclear antigen (PCNA) is a nuclear marker. Tubulin is a cytoplasmic marker. Full size image Further, we applied a biotin–avidin pulldown system to test whether miR-539 could pull down CARL. Cardiomyocytes were transfected with biotinylated miR-539, then harvested for biotin-based pulldown assay. CARL was pulled down as analysed by qRT-PCR, but the introduction of mutations that disrupt base pairing between CARL and miR-539 ( Fig. 6d ) led to the inability of miR-539 to pull down CARL ( Fig. 6e ), indicating that miR-539 recognize CARL is in a sequence-specific manner. In addition, PHB2 was also pulled down by biotinylated miR-539 analysed by qRT-PCR ( Supplementary Fig. 5f ). We also used inverse pulldown assay to test whether CARL could pull down miR-539, a biotin-labelled-specific CARL probe was used. miR-539 was co-precipitated as analysed by the northern blot ( Fig. 6f ). Further, we detected the subcellular location of CARL and miR-539. It showed that CARL was expressed both in nucleus and cytoplasm, and miR-539 was mainly expressed in cytoplasm ( Fig. 6g ). So we applied the biotin-labelled-specific CARL probe to assay where the interaction between CARL and miR-539 is. The results showed that miR-539 could be co-precipitated with CARL in the cytoplasm, but not the nucleus ( Fig. 6h,i ). Taken together, it appears that CARL is able to directly bind to miR-539 in vivo and their interaction is in the cytoplasm. CARL regulates fission and apoptosis through miR-539 and PHB2 As CARL interacts with miR-539, we then tested whether CARL was able to regulate PHB2, which is also the downstream target of miR-539. Knockdown of CARL reduced PHB2 levels in mitochondria ( Fig. 7a ). Overexpression of CARL ( Supplementary Fig. 6a ) resulted in upregulation of PHB2 expression ( Fig. 7b ). CARL counteracted the inhibitory effect of miR-539 on PHB2 expression ( Supplementary Fig. 6b and Fig. 7c ). These results indicated that CARL may act as endogenous sponge ‘antagomir’ of miR-539. 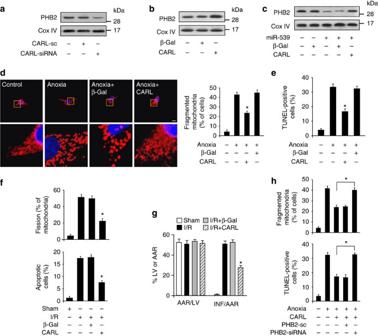Figure 7: CARL regulates mitochondrial fission and apoptosis through targeting miR-539 and PHB2. (a) Knockdown of CARL reduces the expression levels of PHB2 in mitochondria. Cardiomyocytes were infected with adenoviral CARL-siRNA or CARL-sc. Twenty-four hours after infection PHB2 levels in mitochondria were analysed by immunoblot. (b) Enforced expression of CARL induces the increase of PHB2 levels in mitochondria. Cardiomyocytes were infected with adenoviral CARL or β-gal. Twenty-four hours after infection PHB2 levels in mitochondria were analysed. (c) CARL reduces the inhibitory effect of miR-539 on PHB2 expression. Cardiomyocytes were infected with adenoviral miR-539, CARL or β-gal. The levels of PHB2 in mitochondria were analysed by immunoblot. (d,e) CARL inhibits mitochondrial fission and apoptosis induced by anoxia. Cardiomyocytes were infected with adenoviral CARL or β-gal, and then were exposed to anoxia. Mitochondrial fission (d) and apoptosis (e) were assessed. Data are shown as mean±s.e.m. of four independent experiments. *P<0.05 versus anoxia alone in one-way analysis of variance. (f) CARL could inhibit mitochondrial fission and apoptosis upon I/R. Intracoronary delivery of adenoviral constructs of CARL or β-gal and I/R were performed as described in the section of Methods. Counting of fragmented mitochondria and apoptosis were shown. Data are shown as mean±s.e.m. of six independent experiments. *P<0.05 versus I/R alone in one-way analysis of variance. (g) CARL attenuates myocardial INF upon I/R. Mice were treated as described inf. The infarct sizes were shown. Data are shown as mean±s.e.m. of six independent experiments. *P<0.05 versus I/R alone in one-way analysis of variance. (h) Knockdown of PHB2 attenuates the inhibitory effect of CARL on mitochondria fission and apoptosis. Cardiomyocytes were infected with the adenoviral CARL, PHB2-siRNA or PHB2-sc, and then treated with anoxia. Mitochondria fission (upper panel) and apoptosis (low panel) were analysed. Data are shown as mean±s.e.m. of three independent experiments. *P<0.05 in one-way analysis of variance. Figure 7: CARL regulates mitochondrial fission and apoptosis through targeting miR-539 and PHB2. ( a ) Knockdown of CARL reduces the expression levels of PHB2 in mitochondria. Cardiomyocytes were infected with adenoviral CARL-siRNA or CARL-sc. Twenty-four hours after infection PHB2 levels in mitochondria were analysed by immunoblot. ( b ) Enforced expression of CARL induces the increase of PHB2 levels in mitochondria. Cardiomyocytes were infected with adenoviral CARL or β-gal. Twenty-four hours after infection PHB2 levels in mitochondria were analysed. ( c ) CARL reduces the inhibitory effect of miR-539 on PHB2 expression. Cardiomyocytes were infected with adenoviral miR-539, CARL or β-gal. The levels of PHB2 in mitochondria were analysed by immunoblot. ( d , e ) CARL inhibits mitochondrial fission and apoptosis induced by anoxia. Cardiomyocytes were infected with adenoviral CARL or β-gal, and then were exposed to anoxia. Mitochondrial fission ( d ) and apoptosis ( e ) were assessed. Data are shown as mean±s.e.m. of four independent experiments. * P <0.05 versus anoxia alone in one-way analysis of variance. ( f ) CARL could inhibit mitochondrial fission and apoptosis upon I/R. Intracoronary delivery of adenoviral constructs of CARL or β-gal and I/R were performed as described in the section of Methods. Counting of fragmented mitochondria and apoptosis were shown. Data are shown as mean±s.e.m. of six independent experiments. * P <0.05 versus I/R alone in one-way analysis of variance. ( g ) CARL attenuates myocardial INF upon I/R. Mice were treated as described in f . The infarct sizes were shown. Data are shown as mean±s.e.m. of six independent experiments. * P <0.05 versus I/R alone in one-way analysis of variance. ( h ) Knockdown of PHB2 attenuates the inhibitory effect of CARL on mitochondria fission and apoptosis. Cardiomyocytes were infected with the adenoviral CARL, PHB2-siRNA or PHB2-sc, and then treated with anoxia. Mitochondria fission (upper panel) and apoptosis (low panel) were analysed. Data are shown as mean±s.e.m. of three independent experiments. * P <0.05 in one-way analysis of variance. Full size image Enforced expression of CARL ( Supplementary Fig. 6c ) significantly influenced the expression of miR-539 and PHB2 under anoxia condition ( Supplementary Fig. 6d,e ) and inhibited mitochondrial fission ( Fig. 7d ) and apoptosis ( Fig. 7e and Supplementary Fig. 6f ). In the animal model, administration of CARL significantly elevated the levels of CARL ( Supplementary Fig. 7a ), and the overexpressed levels were similar to that in vitro experiment ( Supplementary Fig. 7b ). Enforced expression of CARL ( Supplementary Fig. 7c ) significantly influenced the levels of miR-539 and PHB2 in response to I/R ( Supplementary Fig. 7d, e ), and thus attenuated mitochondrial fission and cell death ( Fig. 7f ), and myocardial INF sizes as well ( Fig. 7g ). Taken together, it appears that CARL is able to prevent mitochondrial fission, apoptosis and myocardial INF. Then, we further tested whether PHB2 is a mediator of CARL. To confirm the relationship between CARL and PHB2 in mitochondrial fission machinery, we knocked down the endogenous PHB2 by PHB2-siRNA construct, and observed that the inhibitory effect of CARL on mitochondrial fission and apoptosis was decreased in the absence of PHB2 ( Supplementary Fig. 7f and Fig. 7h ). Taken together, these data suggest that CARL targets miR-539/PHB2 in the cascades of mitochondrial fission and apoptosis. Mitochondria are highly dynamic structures that fuse and divide continuously to adjust the shape and distribution of the mitochondrial network depending on energy demands. The homeostasis of mitochondrial dynamics is a prerequisite for the maintenance of normal cell metabolism. Here we present evidence for a critical role of PHB2 in regulating mitochondrial dynamics. PHB2 is downregulated in response to the pathological insults, and PHB2 can inhibit mitochondrial fission and apoptosis. In addition, we found that miR-539 is responsible for the downregulation of PHB2, and modulation of miR-539 levels also affects mitochondrial dynamics and apoptosis. Our study further revealed that CARL directly binds to miR-539 and inhibits mitochondrial fission and apoptosis, and this inhibitory effect on mitochondrial fission and apoptosis is dependent on miR-539 and PHB2. Our results provide novel evidence, demonstrating that CARL, miR-539 and PHB2 constitute an axis in the machinery of mitochondrial network. Prohibitins are ubiquitous, evolutionarily conserved proteins that are mainly localized in mitochondria. PHB2 has a predominantly mitochondrial function and it is related to mitochondrial network and apoptosis [26] . Deletion of PHB2 leads to an aberrant cristae morphogenesis and an impaired cellular proliferation and resistance towards apoptosis [14] . This suggests that PHB2 may have an important role in regulating mitochondrial morphology. However, the molecular regulation of PHB2 is poorly understood. Our present work showed that PHB2 expression levels in mitochondria are reduced in response to anoxia and I/R. Overexpression of PHB2 resulted in a reduction in mitochondrial fission and apoptosis. These data suggest that PHB2 can inhibit mitochondrial fission and apoptosis, and PHB2 may antagonize myocardial injury. Previous reports have shown that loss of prohibitins results in the fragmentation of the mitochondrial network in HeLa cells and MEFs [13] , [14] . The mitochondrial fragmentation of PHB2-depleted MEFs strikingly resembles the mitochondrial morphology observed after OPA1 downregulation [14] , [27] . OPA1 is a large dynamin-like GTPase that is found in the mitochondrial intermembrane space and that regulates both mitochondrial fusion and cristae morphogenesis [28] . The aberrant mitochondrial morphology observed in PHB2-depleted MEFs may be explained by an altered processing of OPA1 (ref. 14) [14] . Thus, the results in our present study showing that PHB2 regulates mitochondrial fission cannot exclude an indirect effect of PHB2 upon other mitochondrial functions or oxidative stress. It is also an interesting topic and we will focus on that in our future research. Furthermore, in other cell types, PHB2 has also been suggested to be localized in the nucleus and modulate transcriptional activity by interacting with transcription factors, including nuclear receptors, either directly or indirectly [12] , [29] , [30] , [31] , [32] . PHB2 has been shown to interact with and inhibit the transcriptional activity of the ER in breast cancer [12] . In HeLa cells, mitochondrial PHB2 translocates to the nucleus in the presence of ERα and E2 (ref. 32) [32] . These findings suggest the involvement of mammalian PHB2 protein in the regulation of transcription in the nucleus. In this study, we analysed the mitochondrial PHB2 protein in cardiomyocytes and identified CARL and miR-539 as two novel regulators for PHB2. Further investigations into the function and molecular regulation of PHB2 in mitochondria and nucleus should constitute an important area for future research. Our results may have important therapeutic implications for the employment of PHB2 in the treatment of apoptosis-related diseases. miRNAs have been reported to regulate apoptosis in cardiomyocytes [33] , [34] , [35] . More than 800 miRNAs have been identified. It is critical to identify those miRNAs that are able to regulate apoptosis in the heart and to characterize their signal transduction pathways in the apoptotic cascades. Our present work for the first time demonstrated that miR-539 can regulate mitochondrial fission and apoptosis both in vitro and in vivo through targeting PHB2. Accordingly, it can be speculated that the identification of miRNAs that regulate apoptotic proteins may fill in the gap between unknown aspects of cell biology and the pathogenesis of diseases. LncRNAs have been defined to have important functions in specific cell types, tissues and developmental conditions such as chromatin modification [21] , RNA processing [18] , structural scaffolds [36] , and modulation of apoptosis and invasion and so on [19] . Despite the biological importance of lncRNAs, it is not yet clear whether lncRNAs are involved in the regulation of mitochondrial network. Our present work for the first time reveals a novel function of lncRNA participating in regulating mitochondrial dynamics and myocardial INF, and modulation of its level may provide a new approach for tackling myocardial INF. A recent report showed that a muscle-specific lncRNA, linc-MD1, governs the time of muscle differentiation by acting as a competing endogenous RNA in mouse and human myoblasts [22] . Highly upregulated liver cancer may act as an endogenous ‘sponge’ that downregulates miR-372 leading to reducing translational repression of its target gene, PRKACB [24] . Consistent with these reports, our results suggest that CARL acts as an endogenous sponge for miR-539, thereby regulating the expression of PHB2 that inhibits mitochondrial fission and apoptosis. The discovery of a lncRNA in regulating mitochondrial dynamics by targeting miRNA may shed new lights on understanding the complex molecular mechanism of mitochondrial network. The function of the heart stringently depends on the ATP-generating pathways [37] , and it is therefore enriched in mitochondria. Cardiomyocytes are a good model to study mitochondrial fission because of the abundance of mitochondria. Hitherto, few reports have shown that the abnormal mitochondrial network has a role in the pathogenesis of cardiac diseases. The involvement of lncRNA, miR-539 and PHB2 in regulating mitochondrial networks are revealed in our present study and shed new lights on the understanding of mitochondrial integrity and cardiac pathophysiology. In summary, our present study reveals that miR-539 is integrated into the machinery of mitochondrial dynamics, and that miR-539 can affect mitochondrial apoptotic pathway through targeting PHB2. Moreover, we demonstrated that CARL acts as endogenous sponge RNA and inhibits miR-539 expression and its biological function. Thus, modulation of CARL may represent a novel approach for interventional treatment of heart disease. This finding may provide a new clue for the understanding of lncRNA-controlled cellular events. Cardiomyocytes culture and treatment Cardiomyocytes were isolated from male mice (1–2 days) as we described [38] . Briefly, after dissection hearts were washed and minced in HEPES-buffered saline solution. Tissues were then dispersed in a series of incubations at 37 °C in HEPES-buffered saline solution containing 1.2 mg ml −1 pancreatin and 0.14 mg ml −1 collagenase. Subsequent supernatants were collected and centrifuged at 200 g for 5 min. After centrifugation, cells were re-suspended in Dulbecco’s modified Eagle medium/F-12 (Gibco) containing 5% heat-inactivated horse serum, 0.1 mM ascorbate, insulin-transferring sodium selenite media supplement (Sigma, St. Louis, MO, USA), 100 U ml −1 penicillin, 100 μg ml −1 streptomycin and 0.1 mM bromodeoxyuridine. The dissociated cells were pre-plated at 37 °C for 1 h. The cells were then diluted to 1 × 10 6 cells ml −1 and plated in 10 μg ml −1 laminin-coated different culture dishes according to the specific experimental requirements. Anoxia was performed as we described elsewhere [39] . Briefly, cells were placed in an anoxic chamber with a water-saturated atmosphere composed of 5% CO 2 and 95% N 2 . Apoptosis assays Apoptosis was determined by the terminal deoxyribonucleotidyl transferase-mediated terminal deoxyribonucleotidyl transferase mediated dUTP-digoxigenin nick end labeling (TUNEL) using a kit from Roche. The detection procedures were in accordance with the kit instructions. Caspase-3 was determined by analysing its activity using an Apo-ONE Homogeneous Caspase-3/7 assay kit from Promega according to the manufacturer’s protocol. Target protector preparation Target protector was designed and named as described [23] . In brief, PHB2-TP miR-539 sequence is 5′-GGAGAAATCACATTGTCCCACCCCG-3′. PHB2-TP control sequence is 5′-TGACAAATGAGACTCTCTCCTCTCC-3′. They were synthesized by Gene Tools, and transfected into the cells using the Endo-Porter kit (Gene Tools) according to the kit’s instructions. The target protectors were delivered to the mice by intravenous (i.v.) injection once daily for three consecutive days at 25 mg kg −1 . Immunoblot and immunofluorescence Immunoblot was carried out as we previously described [40] . Briefly, the cells were lysed for 1 h at 4 °C in a lysis buffer (20 mmol l −1 Tris, pH 7.5, 2 mmol l −1 EDTA, 3 mmol l −1 EGTA, 2 mmol l −1 dithiothreitol (DTT), 250 mmol l −1 sucrose, 0.1 mmol l −1 phenylmethylsulfonyl fluoride, 1% Triton X-100) containing a protease inhibitor cocktail. The samples were subjected to 12% SDS-PAGE and transferred to nitrocellulose membranes. Equal protein loading was controlled by Ponceau Red staining of membranes. Blots were probed using the primary antibodies. The anti-PHB2 (1:500) and anti-proliferating cell nuclear antigen (1:1,000) were obtained from Santa Cruz Biotechnology. The anti-COX IV (1:1,000) and anti-tubulin (1:2,000) were obtained from Abcam. After four times washing with PBS, the horseradish peroxidase-conjugated secondary antibodies were added. Antigen–antibody complexes were visualized by enhanced chemiluminescence. Unedited versions of Fig. 7c (PHB2) and (Cox IV) are shown in Supplementary Fig. 8 . Immunofluorescence was performed as we described [40] . The samples were imaged using a laser scanning confocal microscope (Zeiss LSM 510 META). Preparations of subcellular fractions Subcellular fractions were prepared as we described [40] . In brief, the cells were washed twice with PBS and the pellets were suspended in 0.2 ml of buffer A (20 mmol l −1 HEPES, pH 7.5, 10 mmol l −1 KCl, 1.5 mmol l −1 MgCl2, 1 mmol l −1 EGTA, 1 mmol l −1 EDTA, 1 mmol l −1 DTT, 0.1 mmol l −1 phenylmethanesulfonyl fluoride (PMSF) and 250 mmol l −1 sucrose) containing a protease inhibitor cocktail. The cells were homogenized by 12 strokes in a Dounce homogenizer. The homogenates were centrifuged twice at 750 g for 5 min at 4 °C to collect nuclei and debris. The supernatants were centrifuged at 10,000 g for 15 min at 4 °C to collect mitochondria-enriched heavy membrane pellet. The resulting supernatants were centrifuged to yield cytosolic fractions. Pulldown assay with biotinylated miRNA Cardiomyocytes were transfected with biotinylated miRNA (50 nM), harvested 48 h after transfection. The cells were washed with PBS followed by brief vortex and incubated in a lysis buffer (20 mM Tris, pH 7.5, 200 mM NaCl, 2.5 mM MgCl2, 0.05% Igepal, 60 U ml −1 Superase-In (Ambion), 1 mM DTT, protease inhibitors (Roche)) on ice for 10 min. The lysates were precleared by centrifugation and 50 μl of the samples were aliquoted for input. The remaining lysates were incubated with M-280 streptaviden magnetic beads (Sigma). To prevent non-specific binding of RNA and protein complexes, the beads were coated with RNase-free bovine serum albumin (BSA) and yeast tRNA (both from Sigma). The beads were incubated at 4 °C for 3 h, washed twice with ice-cold lysis buffer, three times with the low salt buffer (0.1% SDS, 1% Triton X-100, 2 mM EDTA, 20 mM Tris-HCl, pH 8.0 and 150 mM NaCl), and once with the high salt buffer (0.1% SDS, 1% Triton X-100, 2 mM EDTA, 20 mM Tris-HCl, pH 8.0 and 500 mM NaCl). The bound RNAs were purified using Trizol for the analysis. Pulldown assay with biotinylated DNA probe The biotinylated DNA probe complementary to CARL was synthesized and dissolved in 500 μl of wash/binding buffer (0.5 M NaCl, 20 mM Tris-HCl, pH 7.5, and 1 mM EDTA). The probes were incubated with streptavidin-coated magnetic beads (Sigma) at 25 °C for 2 h to generate probe-coated magnetic beads. Cardiomyocyte lysates were incubated with probe-coated beads, and after washing with the wash/binding buffer, the RNA complexes bound to the beads were eluted and extracted for northern blot analysis. The following primer sequences were used: CARL pulldown probe, 5′-GGGGTCCTGAAGGAAGAGATGGG-3′; and random pulldown probe, 5′-TGATGTCTAGCGCTTGGGCTTTG-3′. Transfection of the antagomirs The chemically modified antagomirs complementary to miR-539 designed to inhibit endogenous miR-539 expression, and the antagomir-negative control (anta-NC) were obtained from GenePharma Co. Ltd. The antagomir sequence was 5′-ACACACCAAGGAUAAUUUCUCC-3′. The anta-NC sequence was 5′-CAGUACUUUUGUGUAGUACAA-3′. Cells were transfected with the antagomirs or the antagomir-NC using Lipofectamine 2000 (Invitrogen) according to the manufacturer’s instruction. Preparations of miR-539 and CARL expression constructs miR-539 was synthesized by PCR using genomic DNA as the template. The forward primer was 5′-GAAGAGGCTAACGTGAGGTTG-3′ and the reverse primer was 5′-CACCATGACCAAGCCACGTAG-3′. CARL was synthesized by PCR using mouse cDNA as the template. The forward primer was 5′-GGACAAACCCCTATAGGCTACT-3′ and the reverse primer was 5′-CTACCAGGATCACTTTCCTTTG-3′. The PCR fragment was finally cloned into the Adeno-X Expression System (Clontech) according to the manufacturer’s instructions. Adenoviral constructions and infection PHB2 was synthesized by PCR using mouse cDNA as the template. The forward primer was 5′-ATGGCCCAGAACTTGAAGGAC-3′ and the reverse primer was 5′-GGTTCTTGATGTCCACACTCA-3′. The adenoviruses harbouring the PHB2 were constructed using the Adeno-X expression system (Clontech). The adenovirus containing β-gal is as we described elsewhere [41] . The PHB2 RNA interference (siRNA) target sequence is 5′-AGACCTGCAGATGGTGAAC-3′. A scramble form was used as a control, 5′-GACTGACGTAGCATGCAGA-3′. The CARL-siRNA target sequence is 5′-TTAAGAGAAGATAATTAAG-3′. The scramble CARL sequence is 5′-GAATAGATAGATAATGATA-3′. The adenoviruses harbouring PHB2-siRNA or CARL-siRNA were constructed using the pSilencer adeno 1.0-CMV System (Ambion) according to the instructions in the kit. All constructs were amplified in HEK293 cells. Adenoviral infection of cardiomyocytes was performed as we described previously [42] . Quantitative reverse transcription-PCR Stem-loop qRT-PCR for mature miR-539 was performed as described [43] on a CFX96 Real-Time PCR Detection System (Bio-Rad). Total RNA was extracted using Trizol reagent. After DNAse I (Takara, Japan) treatment, RNA was reverse transcribed with reverse transcriptase (ReverTra Ace, Toyobo). The levels of miR-539 analysed by qRT-PCR were normalized to that of U6. U6 primers were forward: 5′-GCTTCGGCAGCACATATACTAA-3′ and reverse: 5′-AACGCTTCACGAATTTGCGT-3′. qRT-PCR for CARL were performed as we described [44] . The sequences of CARL primers were forward: 5′-GCAGAGACGCAGCATATGGTT-3’ and reverse: 5′-TCGGGCCTCTCTAAATCGGGA-3′. The results were standardized to control values of glyceraldehyde-3-phosphate dehydrogenase (GAPDH). GAPDH forward primer: 5′-TGTGTCCGTCGTGGATCTGA-3′ and reverse: 5′-CCTGCTTCACCACCTTCTTGA-3′. The specificity of the PCR amplification was confirmed by agarose gel electrophoresis. Absolute quantification using real-time RT-PCR We measured the absolute copy number using the standard curve method. The cDNA of CARL was cloned into pcDNA 3.1 vector. The vector was linearized and sense RNA transcript was generated using in vitro T7 promoter transcription system (Promega). After digested with RNase-free DNAse and purification, the transcript was quantified on a spectrophotometer and converted to the number of copies using the following formula: copy number per microlitre . The quantified RNA was used as the standard of CARL. Synthetic miR-539 RNA was used as the standard of miR-539. For detection of CARL, the standard and total RNA were reverse transcribed with ReverTra Ace (Toyobo) using the reverse primer. The standard of miR-539 were reverse transcribed the same as endogenous miR-539. The standard cDNA was serially diluted in nuclease-free water. Serial dilutions from 10 6 to 10 1 copies were used for standard in a final volume of 20 μl alongside a NC (RNA) and a non-template control. The SYBR Premix Ex Taq II Kit (Takara) was used for amplification. qPCR was performed on a CFX96 Real-Time PCR Detection System (Bio-Rad). Absolute quantification determines the actual copy numbers of target genes by relating the Ct value to a standard curve. The data were analysed by CFX96 software. The final data was expressed as the copy number per 10 pg of total RNA. Northern blot analysis Northern blot was performed as described [45] . In brief, the samples were run on a 15% polyacrylamide–urea gel, transferred to positively charged nylon membranes (Millipore) followed by cross-linking through UV irradiation. The membranes were subjected to hybridization with 100 pmol 3′-digoxigenin (DIG)-labelled probes overnight at 42 °C. Probes were labelled with DIG using a 3′-End DIG Labeling Kit (Roche). The detection was performed using a DIG luminescent detection kit (MyLab) according to the manufacturer’s instructions. The probe sequence for miR-539 was 5′-ACACACCAAGGATAATTTCTCC-3′. U6 was used as an internal control, and its probe sequence was 5′-GCTAATCTTCTCTGTATCGTTCC-3′. The probe sequence for PHB2-TP miR-539 was 5′-CGGGGTGGGACAATGTGATTTCTCC-3′. The probe sequence for PHB2-TP control was 5′-GGAGAGGAGAGAGTCTCATTTGTCA-3′. Luciferase constructs and transfection PHB2 3′-UTR was amplified by PCR. The forward primer was 5′-TGTGGACATCAAGAACCCCAC-3′. The reverse primer was 5′-TGAGAATTCCTGGCATGGTGG-3′. To produce mutated 3′-UTR, the mutations were generated using QuikChange II XL Site-Directed Mutagenesis Kit (Stratagene). WT and mutated 3′-UTRs were subcloned into the pGL3 vector (Promega) immediately downstream the coding region of luciferase gene. Mouse CARL WT (CARL-wt) and the mutant derivative devoid of miR-539-binding site (CARL-mut) were cloned downstream the coding region of luciferase gene. The forward primer was 5′-GGACAAACCCCTATAGGCTACT-3′ and the reverse primer was 5′-TCGGGCCTCTCTAAATCGGGA-3′. miR-539 sensor reporter was constructed according to the method previously described [24] . Briefly, mouse genomic sequence (200 bp) flanking pre-miR-539 was reversely inserted into the pGL3 vector, downstream of the coding region of luciferase gene. HEK293 cells or cardiomyocytes were infected with the indicated adenoviruses, then transfected with the indicated luciferase constructs as described in the corresponding figure legends. The transfection was performed using Lipofectamine 2000 (Invitrogen) according to the manufacturer’s instruction. The luciferase activity was analysed as we described elsewhere [46] . Mitochondrial staining Mitochondrial staining was carried as we and others described with modifications [4] , [47] . Briefly, cells were plated onto the coverslips coated with 0.01% poly-L-lysine. After treatment, they were stained for 20 min with 0.02 μM MitoTracker Red CMXRos (Molecular Probes). Mitochondria were imaged using a laser scanning confocal microscope (Zeiss LSM 510 META). The percentage of cells with fragmented mitochondria relative to the total number of cells is presented as the mean±s.e.m. of at least three independent experiments, counted by an observer blinded to the experimental conditions. Six distinct fields for each 50 cells were counted. At least 300 cells per group were counted. Animal experiments Male adult C57BL/6 mice (8 weeks old) were obtained from Institute of Laboratory Animal Science of Chinese Academy of Medical Sciences (Beijing, China). All experiments were performed according to the protocols approved by the Animal Care Committee, Institute of Zoology, Chinese Academy of Sciences. For intracoronary delivery of adenoviruses, the mice were anaesthetized and ventilated with a HX-300S animal ventilator. The chest was entered through a small left anterior thoracotomy, the pericardial sac was then removed, and 2 × 10 10 moi adenoviruses of PHB2, 2 × 10 10 moi adenoviruses of PHB2-siRNA or 2 × 10 11 moi adenoviruses of CARL were injected with a catheter from the apex of the left ventricle (LV) into the aortic root while the aorta and pulmonary arteries were cross-clamped. The clamp was maintained for 20 s when the heart pumped against a closed system. After removal of air and blood, the chest was then closed and the mice were returned back to cage for recovery. Five days after the injection of adenoviruses, the mice were subjected to I/R surgery. For miR-539 antagomir delivery, chemically modified antagomirs were 2′-OMe modified (GenePharma, Shanghai). The mice received on three consecutive days, i.v. injections of antagomirs and their controls at doses of 30 mg kg −1 body weight in a small volume (0.2 ml) per injection. The mice were then subjected to I/R surgery. For PHB2 target protectors delivery, the target protectors were delivered to the mice by i.v. injection once daily for three consecutive days at 25 mg kg −1 and the mice were then subjected to I/R surgery. For I/R injury model, mice were subjected to 45 min ischaemia, then 3 h or 1 week reperfusion as described [33] . Sham-operated group experienced the same procedure except the snare was left untied. Evans blue dye (1 ml of a 2.0% solution; Sigma-Aldrich) was injected into jugular vein into the heart for delineation of the ischaemic zone from the nonischemic zone. The heart was rapidly excised. The heart slices were incubated in 1.0% 2,3,5-triphenyltetrazolium chloride (Sigma-Aldrich) for 15 min at 37 °C for demarcation of the viable and nonviable myocardium within the risk zone. The staining was stopped by ice-cold sterile saline and the slices were fixed in 10% neutral-buffered formaldehyde and individually weighed. Both sides of each slice were photographed. The areas of INF, area-at-risk (AAR), and nonischemic LV were assessed with computer-assisted planimetry (NIH Image 1.57) by an observer blinded to the sample identity. The ratio of AAR/LV, INF/AAR and INF/LV were calculated. Ventricular tissues were prepared from two different areas: AAR in the centre of the territory of the left anterior descending coronary artery and the remote area in the posterior part of the LV far from the AAR. The tissues were then washed with cold saline and used for real-time analysis. Echocardiographic assessment Transthoracic echocardiographic analysis was performed on mice after 1 week of the sham or I/R surgery as we described [41] . Echocardiographic parameters such as systolic left ventricular internal diameters and diastolic left ventricular internal diameters were measured. Fractional shortening of left ventricular diameter was shown. After in vivo evaluation of cardiac function, the mice were killed and the hearts were harvested, weighted and used for histological examination. Histology The harvested hearts were fixed in 10% formalin and embedded in paraffin and sectioned at 6 μm thickness. TUNEL staining was performed as manufacturer’s procedure (Roche). Cardiomyocytes were identified by α-actinin and the total nuclei were stained by DAPI. Magnification × 40 photos were taken, and 25 random fields for each heart sample were quantified by an investigator who was blind to the treatment. The results are expressed as mean±s.e.m. for at least three independent experiments. Electron microscopy Heart ultrastructural analyses were performed to quantify mitochondrial fission. Sample preparations and conventional electron microscopy were carried out as described before [33] . Samples were examined at a magnification of 15,000 with a JEOL JEM-1230 transmission electron microscope. For comparison of mitochondrial fission, EM micrographs of thin sections were evaluated. The size of individual mitochondrion was measured by using Image-Pro Plus software. Approximately 1,200–1,500 mitochondria were measured to determine the percentages of mitochondria with various sizes. In I/R-treated heart tissues, mitochondria disintegrated into numerous small round fragments of varying size, the number of small mitochondrion was increasing. Thus, we determined the mitochondria with size less than 0.6 mm 2 as fission mitochondria. Data represent mean±s.e.m. of at least three independent experiments. Statistical analysis Data are expressed as the mean±s.e.m. of at least three independent experiments. We evaluated the data with Student’s t -test. We used a one-way analysis of variance for multiple comparisons. A value of P <0.05 was considered significant. How to cite this article: Wang, K. et al. CARL lncRNA inhibits anoxia-induced mitochondrial fission and apoptosis in cardiomyocytes by impairing miR-539-dependent PHB2 downregulation. Nat. Commun. 5:3596 doi: 10.1038/ncomms4596 (2014).